Calcium-dependent permeabilization of erythrocytes by a perforin-like protein during egress of malaria parasites Clinical malaria is associated with proliferation of blood-stage parasites. During the blood stage, Plasmodium parasites invade host red blood cells, multiply, egress and reinvade uninfected red blood cells to continue the life cycle. Here we demonstrate that calcium-dependent permeabilization of host red blood cells is critical for egress of Plasmodium falciparum merozoites. Although perforin-like proteins have been predicted to mediate membrane perforation during egress, the expression, activity and mechanism of action of these proteins have not been demonstrated. Here, we show that two perforin-like proteins, perforin-like protein 1 and perforin-like protein 2, are expressed in the blood stage. Perforin-like protein 1 localizes to the red blood cell membrane and parasitophorous vacuolar membrane in mature schizonts following its Ca 2+ -dependent discharge from micronemes. Furthermore, perforin-like protein 1 shows Ca 2+ -dependent permeabilization and membranolytic activities suggesting that it may be one of the effector proteins that mediate Ca 2+ -dependent membrane perforation during egress. The clinical symptoms of malaria are directly attributed to the blood stage of malaria parasite infection. In this stage, merozoites invade red blood cells (RBCs), replicate and exit out of host RBCs upon maturation to reinvade uninfected RBCs and continue their life cycle [1] , [2] , [3] , [4] , [5] , [6] . The exit of merozoites from host RBCs following rupture of the parasitophorous vacuolar membrane (PVM) and host RBC membrane (RBCM), a process known as egress, is a critical step in the propagation of blood-stage malaria parasites. A clear understanding of the molecular mechanisms involved in parasite egress from infected RBCs could lead to the development of novel approaches to inhibit egress, limit blood-stage parasite growth and protect against malaria. Egress of P. falciparum merozoites is a highly regulated and active process [5] , [7] , [8] , [9] , [10] , [11] , [12] , [13] , which involves many parasite proteases that mediate rupture of the two limiting membranes, PVM and RBCM [14] , [15] , [16] . Studies using fluorescence resonance energy-transfer peptide substrates have revealed the role of intracellular Ca 2+ in the activation of blood-stage parasite proteases that have a role in egress [17] , [18] . In addition to the parasite proteases, activation of a host cell protease, calpain, by intracellular Ca 2+ is also shown to mediate egress [8] . Recent studies also demonstrate the important role of a calcium-dependent protein kinase 5 and a cGMP-dependent protein kinase in egress of P. falciparum merozoites [9] , [13] . Moreover, the regulation of tachyzoite egress by intracellular Ca 2+ is well established in Toxoplasma gondii [19] , [20] , [21] , [22] , [23] . Apart from proteases, a perforin-like protein (PLP) has been shown to be critical in disruption of the host cell membrane in the related apicomplexan T. gondii [23] . Presence of perforins is reported in various cell types for their unique mode of action in formation of pores resulting in the lysis of the target cell [19] , [20] , [21] , [22] , [23] , [24] , [25] . The functional activity of perforins relies on their central MACPF (membrane attack complex pore forming) domain [21] , [22] , [23] , [26] , [27] , [28] . These proteins, which are usually secreted by the host cell in monomeric form, polymerize on the target cell membrane to create pores [28] , [29] . Pathogens utilize pore-forming proteins for cell invasion, cell transversal and lysis of endosomal vesicles for their release in the host cytosol [30] , [31] , [32] , [33] . In rodents, malaria parasites PLPs were found to have a role in cell traversal of mosquito midgut epithelium by ookinetes and hepatic cells by sporozoites [31] , [32] , [33] . Genes for five PLPs have been annotated in P. falciparum and the expression of all PfPLPs has been detected at transcript level using RNA-Seq technique [34] , [35] , [36] . However, the functional roles of the PfPLPs at different stages of the parasite life cycle have not been elucidated. The current study provides mechanistic insights into the activity of a pore-forming MACPF protein, PfPLP1, and parasite egress. We also show that intracellular Ca 2+ regulates permeabilization of the host RBCM and serves as a signal for egress of P. falciparum merozoites. Two PfPLPs, perforin-like protein 1 and 2 (PfPLP1 and PfPLP2) are expressed in the blood-stage parasites and PfPLP1 localizes to micronemes of merozoites. Our results demonstrate that in mature schizonts, intracellular Ca 2+ triggers discharge of PfPLP1 from micronemes. The secreted PfPLP1 binds to membranes in a Ca 2+ -dependent manner. In addition, we demonstrate that Ca 2+ has an essential role in controlling the membranolytic activity of PfPLP1. We also demonstrate that binding of PfPLP1 monomers to RBCMs leads to their oligomerization, which is a pre-requisite step in pore formation by PLPs. These results identify that egress of P. falciparum is regulated by the Ca 2+ -dependent permeabilization of host cell membrane following discharge of PfPLP1 from micronemes. Ca 2+ flux and RBCM permeabilization during merozoite egress To understand the role of Ca 2+ in egress, purified P. falciparum schizonts were loaded with the intracellular Ca 2+ indicator, Fluo-4AM, and observed by time-lapse video microscopy as described earlier [12] , [37] . An increase in intracellular Ca 2+ is observed in schizonts just before egress suggesting that Ca 2+ might have a role in regulating egress of merozoites ( Supplementary Movie 1 ; Fig. 1a ). The rise in intracellular Ca 2+ is crucial as P. falciparum schizonts treated with intracellular Ca 2+ chelator BAPTA-AM (50 μM) showed inhibition of merozoite egress ( Fig. 1c ). Chelation of extracellular Ca 2+ by EGTA (1 mM) has no effect on egress of P. falciparum merozoites as reported previously [12] . Schizonts were also treated with 10 μM cysteine protease inhibitor E64 as a control for inhibition of egress. Both E64 and BAPTA-AM showed 60–70% inhibition in egress ( Fig. 1c ). The treatment of schizonts with BAPTA-AM and EGTA did not affect the viability of the parasite as analysed by staining with Dihydroethidium staining (DHT) ( Fig. 1d ). 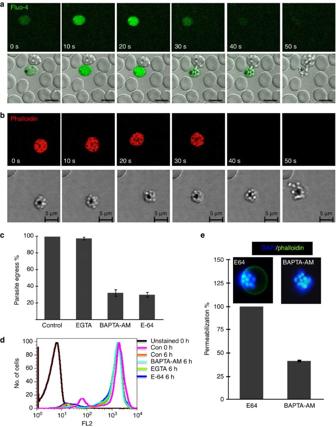Figure 1: Intracellular Ca2+and host cell membrane permeabilization during egress of merozoites. (a) Intracellular Ca2+levels were monitored inP. falciparumschizonts loaded with Ca2+indicator dye, Fluo-4AM, by time-lapse video microscopy. An increase in intracellular Ca2+was observed just before egress. Selected frames of fluorescent images and DIC images merged with fluorescence images with time elapsed between frames are shown. Black bar indicates 5 μm. SeeSupplementary Movie 1. (b) Host cell membrane permeabilization was monitored by time-lapse video microscopy in the presence of 100 μM Phalloidin Alexa 594. Phalloidin staining, indicating permeabilized host cell membrane, was observed just before egress. Selected frames of DIC and fluorescence images of Phalloidin with time elapsed between frames are shown. Scale bar, 5 μm. SeeSupplementary Movie 2. (c) Effect of intracellular Ca2+on egress. Mature schizonts were treated with extracellular Ca2+chelator EGTA, intracellular Ca2+chelator BAPTA-AM and cysteine protease inhibitor E64 in cRPMI for 1 h. Number of schizonts with respect to initial number of schizonts were counted by flow cytometry and percentage of ruptured schizonts was plotted as per cent egress. BAPTA-AM- and E64-treated schizonts show 60–70% inhibition in egress as compared with cRPMI control and EGTA. (d) Viability of schizonts after treatments were analyzed by Flow cytometer following staining with DHT. (e) Regulation of host cell membrane permeabilization by intracellular Ca2+. Permeabilization of BAPTA-AM and E64-treated schizonts was measured by flow cytometry using Phalloidin. The schizonts were also visualized for Phalloidin Alexa 488 staining under fluorescence microscope as shown in the inset. Phalloidin Alexa 488 staining (green) was not detected in BAPTA-AM-treated schizonts. Nuclei were counterstained with DAPI. Figure 1: Intracellular Ca 2+ and host cell membrane permeabilization during egress of merozoites. ( a ) Intracellular Ca 2+ levels were monitored in P. falciparum schizonts loaded with Ca 2+ indicator dye, Fluo-4AM, by time-lapse video microscopy. An increase in intracellular Ca 2+ was observed just before egress. Selected frames of fluorescent images and DIC images merged with fluorescence images with time elapsed between frames are shown. Black bar indicates 5 μm. See Supplementary Movie 1 . ( b ) Host cell membrane permeabilization was monitored by time-lapse video microscopy in the presence of 100 μM Phalloidin Alexa 594. Phalloidin staining, indicating permeabilized host cell membrane, was observed just before egress. Selected frames of DIC and fluorescence images of Phalloidin with time elapsed between frames are shown. Scale bar, 5 μm. See Supplementary Movie 2 . ( c ) Effect of intracellular Ca 2+ on egress. Mature schizonts were treated with extracellular Ca 2+ chelator EGTA, intracellular Ca 2+ chelator BAPTA-AM and cysteine protease inhibitor E64 in cRPMI for 1 h. Number of schizonts with respect to initial number of schizonts were counted by flow cytometry and percentage of ruptured schizonts was plotted as per cent egress. BAPTA-AM- and E64-treated schizonts show 60–70% inhibition in egress as compared with cRPMI control and EGTA. ( d ) Viability of schizonts after treatments were analyzed by Flow cytometer following staining with DHT. ( e ) Regulation of host cell membrane permeabilization by intracellular Ca 2+ . Permeabilization of BAPTA-AM and E64-treated schizonts was measured by flow cytometry using Phalloidin. The schizonts were also visualized for Phalloidin Alexa 488 staining under fluorescence microscope as shown in the inset. Phalloidin Alexa 488 staining (green) was not detected in BAPTA-AM-treated schizonts. Nuclei were counterstained with DAPI. Full size image To study host cell membrane permeabilization during egress, time-lapse video microscopy experiments were performed with mature schizonts in the presence of Phalloidin Alexa 594, which stains actin in permeabilized cells [10] . Phalloidin showed staining of RBCM of schizonts before egress suggesting that host cell membrane permeabilization precedes egress of P. falciparum merozoites ( Supplementary Movie 2 ; Fig. 1b ). Furthermore, host cell membrane permeabilization in BAPTA-AM- and E64-treated schizonts was measured by flow cytometry using Phalloidin Alexa 488 ( Fig. 1e ). Phalloidin Alexa 488 staining could be seen in E64-treated schizonts but not in BAPTA-AM-treated schizonts, suggesting that chelation of intracellular Ca 2+ inhibits RBCM permeabilization. PfPLPs show high degree of homology to known perforins A search of the P. falciparum database for the presence of MACPF domain-containing proteins revealed presence of five PfPLPs. All five PfPLPs possess a N-terminal signal sequence, a MACPF domain and a C-terminal β sheet rich domain ( Fig. 2a ). N-terminal region of PfPLPs show least homology within the family in terms of length and amino-acid sequence. 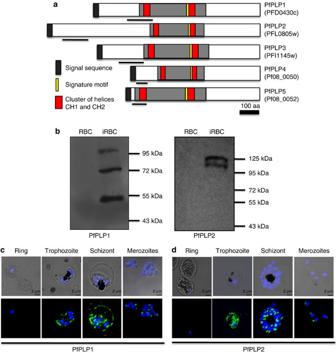Figure 2: Protein architecture and expression profile of different PfPLPs. (a) Schematic representation of all PfPLPs (PfPLP1 (PFD0430c), PfPLP2 (PFL0805w), PfPLP3 (PFI1145w), PfPLP4 (Pf08_0050) and PfPLP5 (Pf08_0052)). The signal sequence (dark grey box) and MACPF (Membrane attack complex/Perforin) domain (Light grey box) are represented. The MACPF domain includes a conserved signature motif (shown in yellow box), and two transmembrane helical domains, CH1 and CH2 (shown in red boxes). The region underlined denotes the region of the protein against which antibodies have been raised. Scale bar, 100 aa. (b) Expression of PfPLPs in the blood stage ofP. falciparum. P. falciparumculture containing rings, trophozoites and schizonts (iRBC) was saponin treated, lysed and probed with antisera of different PfPLPs by western blotting. PfPLP1 and PfPLP2 were detected in the western blot corresponding to the full-length size of ~95 and ~125 kD respectively. RBC lysate was also probed with antisera of PfPLP’s as a negative control. (c,d) Stage-specific expression of PfPLP1 and PfPLP2 in the blood stage ofP. falciparum. Expression of PfPLP1 and PfPLP2 starts in trophozoite stage, with maximal expression in schizonts. In mature schizonts, PfPLP1 and PfPLP2 show punctate staining at the apical end of merozoites. PfPLP1 also shows a ring-like staining, suggesting its localization to RBCM. Scale bar, 2 μm. Figure 2: Protein architecture and expression profile of different PfPLPs. ( a ) Schematic representation of all PfPLPs (PfPLP1 (PFD0430c), PfPLP2 (PFL0805w), PfPLP3 (PFI1145w), PfPLP4 (Pf08_0050) and PfPLP5 (Pf08_0052)). The signal sequence (dark grey box) and MACPF (Membrane attack complex/Perforin) domain (Light grey box) are represented. The MACPF domain includes a conserved signature motif (shown in yellow box), and two transmembrane helical domains, CH1 and CH2 (shown in red boxes). The region underlined denotes the region of the protein against which antibodies have been raised. Scale bar, 100 aa. ( b ) Expression of PfPLPs in the blood stage of P. falciparum. P. falciparum culture containing rings, trophozoites and schizonts (iRBC) was saponin treated, lysed and probed with antisera of different PfPLPs by western blotting. PfPLP1 and PfPLP2 were detected in the western blot corresponding to the full-length size of ~95 and ~125 kD respectively. RBC lysate was also probed with antisera of PfPLP’s as a negative control. ( c , d ) Stage-specific expression of PfPLP1 and PfPLP2 in the blood stage of P. falciparum . Expression of PfPLP1 and PfPLP2 starts in trophozoite stage, with maximal expression in schizonts. In mature schizonts, PfPLP1 and PfPLP2 show punctate staining at the apical end of merozoites. PfPLP1 also shows a ring-like staining, suggesting its localization to RBCM. Scale bar, 2 μm. Full size image The MACPF domains of PfPLPs exhibit core sequence elements; a signature motif (Y/W)-X6-(F/Y)GTH(F/Y)-X6-GG and two transmembrane helices (CH1 and CH2) that are predicted to have an important role in pore formation ( Fig. 2a ). Phylogenetic analysis and ClustalW sequence alignment of MACPF domains of apicomplexan PLPs, human perforin and Photorhabdus luminescens perforin [38] (a MACPF domain-containing protein from a pathogen for which crystal structure has been solved) revealed that PfPLPs are closely related to the human perforin and T. gondii PLP1 (TgPLP1) ( Supplementary Figs S1 and S2 ). Furthermore, in silico modelling of MACPF domains of PfPLPs based on lymphocyte perforin structure [39] (PDB ID 3NSJ) showed significant preservation of the MACPF domain fold with transmembrane helices present on either side of the β-pleated sheet ( Supplementary Fig. S3a ). Transmembrane helices (CH1 and CH2) showed the characteristic features of alternate hydrophilic and hydrophobic residues, which aids in membrane insertion ( Supplementary Fig. S3b ). PfPLP1 and PfPLP2 are expressed in the blood stage To ascertain whether PfPLPs are expressed in the blood stage, reverse transcriptase-PCR analysis was performed in tightly synchronized rings, trophozoites and schizonts of P. falciparum . Transcripts for PfPLP1, PfPLP2, PfPLP3 and PfPLP5 but not PfPLP4 were detected in P. falciparum blood stage ( Supplementary Fig. S4 ). Transcripts for 18S RNA were used as a loading control for RNA from different stages. Primers specific to an intron of PfPLP1 and gametocyte protein, Pfg377, were used in reverse transcriptase-PCR analysis with complementary DNA of different stages as negative controls ( Supplementary Fig. S4 ). To evaluate the expression of PfPLPs at the protein level, P. falciparum lysates containing all the stages, that is, rings, trophozoites and schizonts were probed by western blotting using antibodies specific to each PfPLP ( Supplementary Fig. S5 ). Anti-PfPLP1 and anti-PfPLP2 mouse sera recognized proteins of ~92 and ~122 kDa in the lysate corresponding to their full-length polypeptides, respectively ( Fig. 2b ). Apart from the full-length PfPLP1 and PfPLP2 proteins, truncated polypeptides of ~80 kDa and ~55 kDa were detected by anti-PfPLP1 and a peptide of ~110 kDa was detected by anti-PfPLP2 mouse sera ( Fig. 2b ). The protease PfSUB1 has been predicted to cleave PfPLP1 and PfPLP2 (ref. 14 ) ( Supplementary Fig. S6 ). Anti-PfPLP1 and anti-PfPLP2 mouse sera detect truncated polypeptides of the predicted sizes by western blotting of P. falciparum blood-stage parasite lysates ( Fig. 2b ; Supplementary Fig. S6 ). Western blotting of the lysate with anti-PfPLP3, anti-PfPLP4, anti-PfPLP5, pre-immune sera and anti-GST mouse sera did not detect any protein band (data not shown). To investigate the stage-specific expression of PfPLP1 and PfPLP2, immunofluorescence assay (IFA) was performed using anti-PfPLP1 and anti-PfPLP2 mouse sera with rings, trophozoites, schizonts and merozoites. PfPLP1 and PfPLP2 are detected in late trophozoites, schizonts and merozoites but not in rings by IFA suggesting that expression of PfPLP1 and PfPLP2 is initiated in the late trophozoite stage and increases in mature schizonts and merozoites ( Fig. 2c ). In addition, no staining was observed in any stages with anti-PfPLP3, anti-PfPLP4 and anti-PfPLP5, suggesting that they are not expressed in the blood stage (data not shown). Both PfPLP1 and PfPLP2 show punctate staining in schizonts and apical localization in merozoites. In addition, PfPLP1 is found associated with the RBCM in mature schizonts ( Figs 2c and 3 ), whereas PfPLP2 is not found to localize to RBCM as well as PVM ( Fig. 2d ; Supplementary Figs S7 and S8 ). PfPLP1 might thus have a predominant role in RBCM permeabilization during egress. 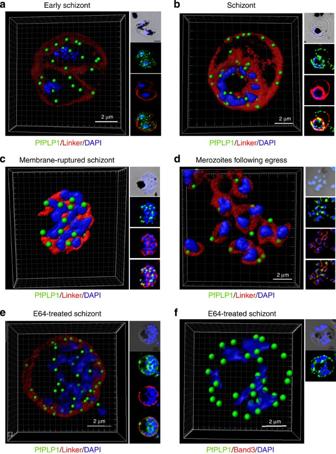Figure 3: Change in localization of PfPLP1 to host cell membrane during egress of merozoites. (a–d) Schizonts were stained with anti-PfPLP1 followed by anti-mouse Alexa-Fluor 488 (green) and membrane-specific linker dye (red) at different time points (~44–48 hpi) during egress. Three-dimensional reconstruction of confocal z-stack images of schizonts was done using Imaris software. PfPLP1 is represented as green dots and membrane dye is shown as two concentric rings corresponding to RBCM and PVM in red. The insets show a bright field and single-slice images with deconvolution. (a) Early schizonts do not show PfPLP1 on the two limiting membranes but shows punctate staining within parasite. (b) Mature schizonts show ring-like staining of PfPLP1 that colocalizes with the membrane dye, suggesting its presence on the membrane. (c) Upon rupture, linker stains the merozoite cell membrane and PfPLP1 shows punctate staining in merozoites with linker staining its cell membrane. (d) After egress, free merozoites show apical localization of PfPLP1. (e,f) Localization of PfPLP1 in E64-treated schizonts. (e) PfPLP1 colocalizes with linker in E64-treated schizonts suggesting that PfPLP1 localizes to PVM in schizonts. (f) E64-treated schizonts did not show staining with anti-band3 antibody where PfPLP1 showed ring-like staining suggestive of its presence on the membrane. Nuclei were counterstained with DAPI. Scale bar, 2 μm. Figure 3: Change in localization of PfPLP1 to host cell membrane during egress of merozoites. ( a–d ) Schizonts were stained with anti-PfPLP1 followed by anti-mouse Alexa-Fluor 488 (green) and membrane-specific linker dye (red) at different time points (~44–48 hpi) during egress. Three-dimensional reconstruction of confocal z-stack images of schizonts was done using Imaris software. PfPLP1 is represented as green dots and membrane dye is shown as two concentric rings corresponding to RBCM and PVM in red. The insets show a bright field and single-slice images with deconvolution. ( a ) Early schizonts do not show PfPLP1 on the two limiting membranes but shows punctate staining within parasite. ( b ) Mature schizonts show ring-like staining of PfPLP1 that colocalizes with the membrane dye, suggesting its presence on the membrane. ( c ) Upon rupture, linker stains the merozoite cell membrane and PfPLP1 shows punctate staining in merozoites with linker staining its cell membrane. ( d ) After egress, free merozoites show apical localization of PfPLP1. ( e , f ) Localization of PfPLP1 in E64-treated schizonts. ( e ) PfPLP1 colocalizes with linker in E64-treated schizonts suggesting that PfPLP1 localizes to PVM in schizonts. ( f ) E64-treated schizonts did not show staining with anti-band3 antibody where PfPLP1 showed ring-like staining suggestive of its presence on the membrane. Nuclei were counterstained with DAPI. Scale bar, 2 μm. Full size image Detection of PfPLP1 by western blot and mass spectrometry We confirmed the specificity of anti-PfPLP1 mouse sera by western blotting with recombinant full-length protein of PfPLP1 and PfPLP2. Anti-PfPLP1 mouse sera recognized only recombinant PfPLP1 protein and not PfPLP2, suggesting that this antibody is specific for PfPLP1 ( Supplementary Fig. S9a ). Furthermore, we confirmed the identity of polypeptides detected in P. falciparum schizonts lysate by probing with anti-PfPLP1 mouse sera generated against a KLH-conjugated PfPLP1 peptide following immunoprecipitation. All three polypeptides (~92, ~80 and 55 kDa) were detected, confirming these polypeptides are fragments of PfPLP1 ( Supplementary Fig. S9b ). Furthermore, these polypeptides were excised from the gel and analyzed by matrix-assisted laser desorption/ionization–time of flight (MALDI TOF/TOF). Both the ~72 and ~95 kDa polypeptides were identified by MALDI TOF/TOF analysis ( Supplementary Fig. S9c,d , Supplementary Table S1 ), however ~55 kDa could not be identified because of insufficient quantity and purity achieved following immunoprecipitation. PfPLP1 localizes to RBCM and PVM during egress To investigate the role of PfPLP1 in egress, its localization was probed by IFA in mature schizonts using anti-PfPLP1 mouse sera and a membrane-specific dye, PKH26 Red Fluorescent Cell Linker Dye (Linker). PfPLP1 was found to localize to both limiting membranes, PVM and RBCM, in mature schizonts as evident from the colocalization of PfPLP1 with the two concentric ring-like staining of RBCM and PVM by linker ( Fig. 3 ). PfPLP1 was also found to colocalize with band 3 at the RBCM ( Supplementary Fig. S8b ). The localization of PfPLP1 on PVM was further confirmed in E64-treated schizonts, which were stained by linker dye but not with anti-band 3 antibody ( Supplementary Fig. S8a ). Previous reports indicate that E64-treated schizonts are enclosed only by PVM [7] , [40] , [41] . PfPLP1 staining was found on the membrane of E64-treated schizonts, which was stained by linker dye, but not with anti-band 3 antibodies indicating that PfPLP1 is associated with PVM ( Fig. 3e ). Apart from membrane localization, PfPLP1 also showed punctate staining within the schizonts ( Fig. 3 ). Next, we investigated localization of PfPLP1 at different stages of schizonts before egress of merozoites. PfPLP1 was not detected on the membranes of early stage schizont ( Fig. 3a ) in contrast to its localization found on the membranes of mature schizonts ( Fig. 3b ). In very mature schizonts, where membranes have disintegrated and merozoites were released, PfPLP1 showed apical localization in merozoites ( Fig. 3c ). These results suggest that PfPLP1, which is initially localized in the parasite binds to the RBCM upon discharge. PfPLP1 is localized to the micronemes of merozoites PLPs are known to localize to secretory organelles in various cell types, which allows their regulated discharge to the target cell membrane [27] , [28] . We studied the subcellular localization of PfPLP1 by co-immunostaining with known apical organelle markers, namely, EBA-175 for micronemes [42] and Clag3.1 for rhoptries [43] . Antisera against MSP1 (merozoite surface protein 1; Fig. 4a ) was used as a marker for the merozoite membrane. PfPLP1 was found to colocalize with EBA-175 suggesting the presence of PfPLP1 in micronemes ( Fig. 4d ). PfPLP1 staining did not colocalize with the rhoptry marker Clag3.1 ( Fig. 4c ). 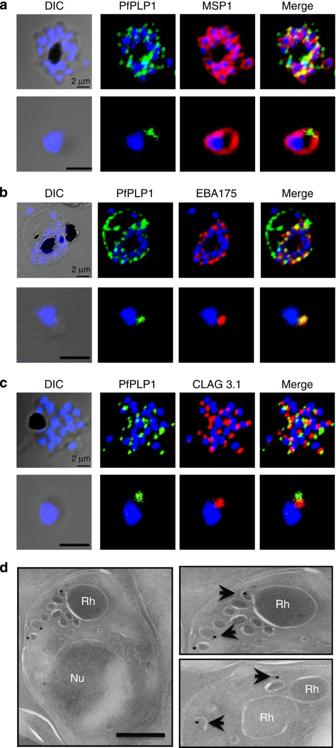Figure 4: Subcellular localization of PfPLP1 in schizonts and merozoites ofP. falciparum. (a) Co-immunostaining of PfPLP1 (green) with merozoite surface protein MSP1 (red). (b) Co-immunostaining of PfPLP1 (green) with micronemal protein EBA-175 (red). PfPLP1 colocalizes with EBA-175 (colocalization coefficient being more than 0.75). (c) Co-immunostaining of PfPLP1 (green) with rhoptry protein CLAG3.1 (red). PfPLP1 is not localized in rhoptry. Nuclei were counterstained with DAPI and Scale bar, 2 μm. (d) Immunoelectron microscopy of PfPLP1. Ultrathin sections of merozoites and late-stage schizonts were labelled with anti-PfPLP1 mouse sera followed by gold-labelled (15 nm) anti-mouse IgG secondary antibodies. Gold particles were detected in elongated, membrane-enclosed micronemes towards the apical end in schizonts and merozoites. Scale bar, 500 nm. Figure 4: Subcellular localization of PfPLP1 in schizonts and merozoites of P. falciparum . ( a ) Co-immunostaining of PfPLP1 (green) with merozoite surface protein MSP1 (red). ( b ) Co-immunostaining of PfPLP1 (green) with micronemal protein EBA-175 (red). PfPLP1 colocalizes with EBA-175 (colocalization coefficient being more than 0.75). ( c ) Co-immunostaining of PfPLP1 (green) with rhoptry protein CLAG3.1 (red). PfPLP1 is not localized in rhoptry. Nuclei were counterstained with DAPI and Scale bar, 2 μm. ( d ) Immunoelectron microscopy of PfPLP1. Ultrathin sections of merozoites and late-stage schizonts were labelled with anti-PfPLP1 mouse sera followed by gold-labelled (15 nm) anti-mouse IgG secondary antibodies. Gold particles were detected in elongated, membrane-enclosed micronemes towards the apical end in schizonts and merozoites. Scale bar, 500 nm. Full size image Immunoelectron microscopy was used to further confirm the localization of PfPLP1. PfPLP1 staining was detected in elongated, membrane-enclosed vesicles towards the apical end confirming its localization to the micronemes of P. falciparum merozoites ( Fig. 4d ). Ca 2+ -dependent discharge and membrane binding of PfPLP1 Membrane localization of PfPLP1 was evaluated in schizonts with and without prior treatment with BAPTA-AM by IFA and western blotting. Unlike untreated schizonts, PfPLP1 was not found on the limiting membranes of BAPTA-AM-treated schizonts. However, it showed punctate staining within merozoites suggesting that PfPLP1 was localized to the micronemes but not secreted in the absence of intracellular Ca 2+ ( Fig. 5a ). The absence of PfPLP1 on the membrane of BAPTA-AM-treated schizonts could be either due to failure of PfPLP1 binding to RBCM in the absence of Ca 2+ or due to inhibition of its secretion from micronemes. 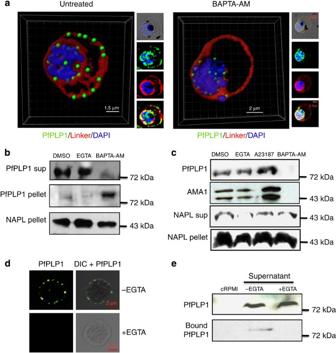Figure 5: Ca2+-dependent discharge and membrane binding of PfPLP1. (a) Membrane localization of PfPLP1 was detected using IFA of untreated and BAPTA-AM-treated schizonts. Schizonts were stained with anti-PfPLP1 (green) and membrane dye (red) and visualized under confocal microscope. Three-dimensional reconstruction from z-stacks of IFA images using Imaris software is shown. PfPLP1 is localized on the RBCM of untreated schizonts but not in BAPTA-AM (B/AM)-treated schizonts, indicating that intracellular Ca2+chelation blocks membrane localization of PfPLP1. (b) Ca2+mediated discharge of PfPLP1 during egress ofP. falciparummerozoites. PV and RBC fraction of schizonts treated with B/AM and EGTA was probed with antisera of PfPLP1. PfPLP1 was not detected in B/AM-treated cells. Parasite pellet was probed with PfPLP1 and NAPL. NAPL serves as loading control. (c) Ca2+-dependent secretion of PfPLP1 fromP. falciparummerozoites. Merozoites were isolated as described earlier37and treated with B/AM, EGTA and Ca2+ionophore A23187. The supernatant of the treated merozoites was probed with antisera of PfPLP1, antisera of AMA1 (microneme protein) and antisera of NAPL (cytoplasmic protein as lysis control) by western blotting. PfPLP1 was secreted in response to ionophore treatment, while its secretion was completely abolished in the presence of B/AM. AMA1, another microneme protein, is a positive control for this experiment. NAPL works as loading control and inadvertent lysis control. iRPMI works as solvent control. (d,e) Ca2+-dependent binding of native PfPLP1. Schizont-ruptured supernatant containing native PfPLP1 was incubated with human RBCs in the presence and absence of EGTA. (d) Human RBCs incubated with schizont-ruptured supernatant in the presence and absence of EGTA were stained with anti-PfPLP1 followed by anti-mouse Alexa-Fluor 488. PfPLP1 staining (green) was seen in the absence of EGTA but not in the presence of EGTA. (e) Western blot analysis of bound PfPLP1 eluted by 1.5 M NaCl. Binding of PfPLP1 was abolished in the absence of Ca2+. Supernatants, before performing EBA, were also probed for native PfPLP1 as a loading control. Figure 5: Ca 2+ -dependent discharge and membrane binding of PfPLP1. ( a ) Membrane localization of PfPLP1 was detected using IFA of untreated and BAPTA-AM-treated schizonts. Schizonts were stained with anti-PfPLP1 (green) and membrane dye (red) and visualized under confocal microscope. Three-dimensional reconstruction from z-stacks of IFA images using Imaris software is shown. PfPLP1 is localized on the RBCM of untreated schizonts but not in BAPTA-AM (B/AM)-treated schizonts, indicating that intracellular Ca 2+ chelation blocks membrane localization of PfPLP1. ( b ) Ca 2+ mediated discharge of PfPLP1 during egress of P. falciparum merozoites. PV and RBC fraction of schizonts treated with B/AM and EGTA was probed with antisera of PfPLP1. PfPLP1 was not detected in B/AM-treated cells. Parasite pellet was probed with PfPLP1 and NAPL. NAPL serves as loading control. ( c ) Ca 2+ -dependent secretion of PfPLP1 from P. falciparum merozoites. Merozoites were isolated as described earlier [37] and treated with B/AM, EGTA and Ca 2+ ionophore A23187. The supernatant of the treated merozoites was probed with antisera of PfPLP1, antisera of AMA1 (microneme protein) and antisera of NAPL (cytoplasmic protein as lysis control) by western blotting. PfPLP1 was secreted in response to ionophore treatment, while its secretion was completely abolished in the presence of B/AM. AMA1, another microneme protein, is a positive control for this experiment. NAPL works as loading control and inadvertent lysis control. iRPMI works as solvent control. ( d , e ) Ca 2+ -dependent binding of native PfPLP1. Schizont-ruptured supernatant containing native PfPLP1 was incubated with human RBCs in the presence and absence of EGTA. ( d ) Human RBCs incubated with schizont-ruptured supernatant in the presence and absence of EGTA were stained with anti-PfPLP1 followed by anti-mouse Alexa-Fluor 488. PfPLP1 staining (green) was seen in the absence of EGTA but not in the presence of EGTA. ( e ) Western blot analysis of bound PfPLP1 eluted by 1.5 M NaCl. Binding of PfPLP1 was abolished in the absence of Ca 2+ . Supernatants, before performing EBA, were also probed for native PfPLP1 as a loading control. Full size image Ca 2+ -dependent secretion of PfPLP1 from micronemes of mature schizonts was assessed by western blotting. Proteins from PV, PVM and RBCM of schizonts treated with either BAPTA-AM, EGTA (extracellular Ca 2+ chelator) or incomplete RPMI, in which similar amount of dimethylsulphoxide (DMSO) used to reconstitute BAPTA-AM is added (DMSO control), were obtained by saponin lysis and probed with anti-PfPLP1 mouse sera. The non-ionic glycoside detergent saponin, at low concentrations permeabilizes both the RBCM and the PVM without disrupting the parasite plasma membrane, thus releasing proteins from PV and RBC [7] , [44] . The processed band of PfPLP1 was detected in saponin-sensitive fraction of untreated and EGTA treated schizonts but not in BAPTA-AM-treated schizonts ( Fig. 5b ), suggesting that chelation of intracellular Ca 2+ blocks secretion of PfPLP1. Presence of PfPLP1 was also probed in the parasite fractions of schizonts treated with BAPTA-AM, EGTA or DMSO control. Higher levels of PfPLP1 were detected in parasite fractions of BAPTA-AM-treated schizonts compared with controls ( Fig. 5b ). Rabbit sera against the cytoplasmic protein NAPL were used as a loading control [37] , [45] . The secretion of PfPLP1 from the micronemes was further tested in free merozoites with and without treatment with BAPTA-AM, EGTA and Ca 2+ ionophore A23187. The secretion of PfPLP1 was found to be triggered by addition of A23187, whereas chelation of intracellular Ca 2+ with BAPTA-AM inhibited secretion of PfPLP1 ( Fig. 5c ). Secretion of microneme protein AMA1 was probed under similar conditions as a control for Ca 2+ -dependent microneme discharge as reported previously [37] . These results suggested that PfPLP1 was secreted from micronemes in a Ca 2+ -dependent manner during egress of P. falciparum merozoites. The binding of native PfPLP1 to human RBCM was tested in the presence and absence of EGTA ( Fig. 5d ) by western blotting and IFA using erythrocyte-binding assays (EBA). Native PfPLP1 bound to RBCM in the presence of Ca 2+ but not in the presence of EGTA (absence of Ca 2+ ), suggesting that Ca 2+ is required for the binding of PfPLP1 to RBCM. Before performing EBA, supernatants were also probed for native PfPLP1 as equal loading controls ( Fig. 5e ). PfPLP1 has potent Ca 2+ -dependent lytic activity To assess the lytic activity of PfPLP1, we expressed full-length PfPLP1 protein (rPfPLP1) and its MACPF (rMACPF) domain in mammalian expression system. Mammalian expression system was advantageous over prokaryotic system for expression of functional PfPLP1 because it possesses a complicated structure and an abundant cysteine-rich domain, which makes it difficult to express in prokaryotic system. rPfPLP1 and rMACPF were expressed as secreted proteins and purified by Ni-NTA chromatography ( Fig. 6a ). Membranolytic activity of rPfPLP1 and rMACPF were tested on human RBCs. rPfPLP1 and rMACPF showed concentration-dependent lysis of human RBCs ( Fig. 6 b ). To test the effect of Ca 2+ on lytic activity of rPfPLP1, lytic assays were performed in the presence and absence of EGTA. Membranolytic activity of rPfPLP1 is detected only in the absence of EGTA, indicating that PfPLP1 requires Ca 2+ for its membranolytic activity ( Fig. 6c ). Membranolytic activity of rMACPF was found to be independent of the presence of Ca 2+ ( Fig. 6 f ). 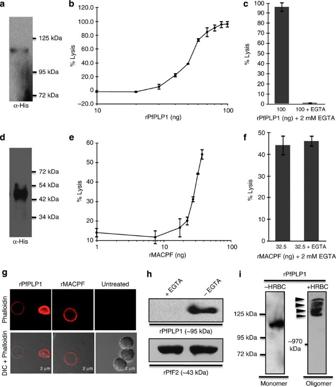Figure 6: Ca2+-dependent permeabilization and membranolytic activity of PfPLP1 (a) Western blot of affinity-purified rPfPLP1 probed with anti-his antibody. (b) Dose-dependent membranolytic activity of recombinant PfPLP1 (rPfPLP1). Lysis of human RBCs was analyzed in the presence of different amount of rPfPLP1. The graph indicates per cent lysis of human RBCs by rPfPLP1 as compared with 100% hypotonic lysis of human RBCs in water. (c) Ca2+-dependent activity of rPfPLP1. The graph shows per cent lysis of human RBC by rPfPLP1 in the presence and absence of EGTA (extracellular Ca2+chelator). Human RBC lysis in the presence of water is used as complete lysis control. (d) Western blot of affinity-purified rMACPF probed with anti-his antibody. (e) Dose-dependent membranolytic activity of rPfPLP1-MACPF. rMACPF domain shows concentration-dependent lytic activity of human RBCs. (f) Ca2+-dependent lytic activity of rPfPLP1-MACPF. rMACPF domain does not show Ca2+-dependent lytic activity. (g) Permeabilization activity of rPfPLP1 and rPfPLP1-MACPF. The human RBCs were incubated with Phalloidin Alexa 594 in the presence and absence of rPfPLP1 and rMACPF and visualized under confocal microscope. Phalloidin staining was detected in the human RBCs treated with rPfPLP1 or rMACPF but not in untreated human RBCs. (h) Western blot analysis of bound rPfPLP1 eluted by 1.5 M NaCl. Binding of rPfPLP1 was abolished in the absence of Ca2+. Recombinant PfF2, the receptor-binding domain of EBA-175, was used as a control for RBC binding. rPfF2 shows Ca2+independent binding to human RBCs. (i) Oligomerization of rPfPLP1. rPfPLP1 is incubated with and without human RBCs at 37 °C for 30 min and analyzed for oligomeric rPfPLP1 by western blotting. Oligomeric PfPLP1 (>1,000 kDa) was detected only upon incubation with human RBC that runs much higher than monomeric PfPLP1, suggesting the presence of more than 15 molecules in the oligomer. Four high-molecular-weight bands were detected (marked by arrow) in the oligomerized fraction indicating heterogeneity of PfPLP1 oligomeric complexes. Figure 6: Ca 2+ -dependent permeabilization and membranolytic activity of PfPLP1 ( a ) Western blot of affinity-purified rPfPLP1 probed with anti-his antibody. ( b ) Dose-dependent membranolytic activity of recombinant PfPLP1 (rPfPLP1). Lysis of human RBCs was analyzed in the presence of different amount of rPfPLP1. The graph indicates per cent lysis of human RBCs by rPfPLP1 as compared with 100% hypotonic lysis of human RBCs in water. ( c ) Ca 2+ -dependent activity of rPfPLP1. The graph shows per cent lysis of human RBC by rPfPLP1 in the presence and absence of EGTA (extracellular Ca 2+ chelator). Human RBC lysis in the presence of water is used as complete lysis control. ( d ) Western blot of affinity-purified rMACPF probed with anti-his antibody. ( e ) Dose-dependent membranolytic activity of rPfPLP1-MACPF. rMACPF domain shows concentration-dependent lytic activity of human RBCs. ( f ) Ca 2+ -dependent lytic activity of rPfPLP1-MACPF. rMACPF domain does not show Ca 2+ -dependent lytic activity. ( g ) Permeabilization activity of rPfPLP1 and rPfPLP1-MACPF. The human RBCs were incubated with Phalloidin Alexa 594 in the presence and absence of rPfPLP1 and rMACPF and visualized under confocal microscope. Phalloidin staining was detected in the human RBCs treated with rPfPLP1 or rMACPF but not in untreated human RBCs. ( h ) Western blot analysis of bound rPfPLP1 eluted by 1.5 M NaCl. Binding of rPfPLP1 was abolished in the absence of Ca 2+ . Recombinant PfF2, the receptor-binding domain of EBA-175, was used as a control for RBC binding. rPfF2 shows Ca 2+ independent binding to human RBCs. ( i ) Oligomerization of rPfPLP1. rPfPLP1 is incubated with and without human RBCs at 37 °C for 30 min and analyzed for oligomeric rPfPLP1 by western blotting. Oligomeric PfPLP1 (>1,000 kDa) was detected only upon incubation with human RBC that runs much higher than monomeric PfPLP1, suggesting the presence of more than 15 molecules in the oligomer. Four high-molecular-weight bands were detected (marked by arrow) in the oligomerized fraction indicating heterogeneity of PfPLP1 oligomeric complexes. Full size image rPfPLP1- and rMACPF-mediated permeabilization of human RBCs is confirmed by performing lysis assay in the presence of Phalloidin Alexa 594. rPfPLP1- and rMACPF-treated human RBCs showed Phalloidin staining suggesting that rPfPLP1 permeabilizes the human RBCs leading to their lysis ( Fig. 6g ). The binding of rPfPLP1 to human RBCM was tested in the presence and absence of Ca 2+ ( Fig. 6h ) by western blotting. rPfPLP1 bound to human RBCs in the presence of Ca 2+ similar to native PfPLP1 ( Fig. 5d ). The receptor-binding domain of erythrocyte-binding antigen (EBA-175), rPfF2, was used as a control in EBA. rPfF2 bound human RBCs, in both, presence and absence of Ca 2+ ( [46] ). As oligomerization of perforins requires membrane binding, the oligomerization of PfPLP1 monomers was evaluated by incubating rPfPLP1 with human RBCs in the presence of Ca 2+ . PfPLP1 was detected in membrane-bound, SDS-resistant, higher-order, membrane-associated fractions suggesting that rPfPLP1 forms oligomers ( Fig. 6i ). Four high-molecular-weight bands present in the oligomer fraction suggests heterogeneity of PfPLP1 oligomeric complexes composed of different number of rPfPLP1 monomers ( Fig. 6i ). Monomers of rPfPLP1 incubated without the human RBCs under similar conditions did not show higher molecular mass complex ( Fig. 6i ). We have investigated the role of intracellular Ca 2+ in the egress of merozoites from P. falciparum- infected RBCs and demonstrated that chelation of intracellular Ca 2+ in schizonts inhibits egress. Furthermore, an increase in intracellular Ca 2+ in schizonts is observed just before egress of merozoites by time-lapse video microscopy ( Fig. 1a ; Supplementary Movie 1 ). Intracellular Ca 2+ , thus appears to have an important role in regulating parasite egress ( Fig. 1c ). We also investigated host cell membrane permeabilization during egress and found that host cell membrane permeabilization precedes egress ( Fig. 1b ; Supplementary Movie 2 ). Chelation of intracellular Ca 2+ in schizonts inhibited permeabilization suggesting that intracellular Ca 2+ has a crucial role in permeabilization of host cell membrane leading to egress ( Fig. 1e ). Host cell membrane permeabilization during egress is mediated by a PLP in T. gondii. The regulation of host cell membrane permeabilization by Ca 2+ may be a result of Ca 2+ -dependent secretion of PfPLP1 from micronemes and its Ca 2+ -dependent membrane binding and lytic activity. The permeabilization of the host cell membrane has been shown to be a pre-requisite step for egress of various apicomplexan parasites, including P. falciparum [10] , [20] , [21] , [22] . PLPs have been studied in rodent malaria parasites and the related apicomplexan parasite T. gondii [23] , [31] , [32] , [33] . While the role of PLPs has been described for invasion of the mosquito midgut epithelium by ookinetes and invasion of hepatocytes by sporozoites, a role for PLPs in the egress of P. falciparum merozoites remains to be described [31] , [32] , [33] . In this study, we demonstrate by western blotting and IFA using specific antisera that two PfPLPs, PfPLP1 and PfPLP2, are expressed in the blood stage of P. falciparum ( Fig. 2b–d ). Of these, we show that PfPLP1 is localized to the two limiting membranes, PVM and RBCM, upon discharge from micronemes of merozoites and binds to RBCM in Ca 2+ -dependent manner ( Figs 3 , 5 and 7 ). 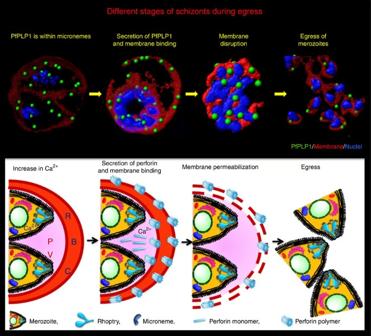Figure 7: Model for PfPLP1-mediated egress. An increase in intracellular Ca2+triggers discharge of PfPLP1 from micronemes of merozoites leading to its localization on the host cell membrane. Localization of PfPLP1 on the membrane mediates its permeabilization and rupture facilitating egress ofP. falciparummerozoites. Figure 7: Model for PfPLP1-mediated egress. An increase in intracellular Ca 2+ triggers discharge of PfPLP1 from micronemes of merozoites leading to its localization on the host cell membrane. Localization of PfPLP1 on the membrane mediates its permeabilization and rupture facilitating egress of P. falciparum merozoites. Full size image Video microscopy observations indicate that merozoite egress is a rapid and tightly regulated event ( Supplementary Movies 1 and 2 ). Regulation of the timing of exit upon schizont maturation is critical as egress of non-invasive and immature merozoites would be disastrous for parasite proliferation. Given the elevated Ca 2+ levels observed in mature schizonts during egress, we investigated whether intracellular Ca 2+ can control this process by regulated secretion of PfPLP1 from micronemes. We tested secretion of PfPLP1 during egress and found that the chelation of intracellular Ca 2+ inhibited PfPLP1 secretion as well as localization onto the host cell membrane of schizonts ( Fig. 5a–c ). Moreover, free merozoites treated with Ca 2+ ionophore A23187 show increased secretion of PfPLP1, whereas BAPTA-AM-treated merozoites do not discharge PfPLP1, confirming that PfPLP1 is secreted from micronemes of merozoites in a Ca 2+ -dependent manner ( Fig. 5c ). Ca 2+ -dependent secretion of PfPLP1 from merozoites ensures increased local concentration on the membrane, which is required to exhibit membranolytic activity just before egress ( Figs 5a,b and 6b ) similar to lymphocyte perforin [28] , [47] , [48] , [49] . Once secreted, PfPLP1 binds the target cell membrane for its activity. We tested the binding of secreted PfPLP1 to RBCM and found that PfPLP1 binds to human RBCs in Ca 2+ -dependent manner ( Figs 5d,e and 6h ). Although apicomplexan PLPs have been shown to be necessary for rapid membrane disruption and appear to have all the necessary structural features for pore formation, their membranolytic activity has not been directly demonstrated by biochemical assays [23] , [31] , [32] , [33] , [50] . We demonstrate the membranolytic activity of PfPLP1 by expressing full-length rPfPLP1 and its rMACPF domain. rPfPLP1 and rMACPF lyse human RBCs in a dose-dependent manner ( Fig. 6b ). rPfPLP1 and rMACPF do not show membranolytic activity at low concentrations suggesting that concentrations above a threshold are required to lyse target cells. This is similar to other MACPF domain-containing proteins [29] , [51] , [52] . This also explains a high concentration requirement of native PfPLP1 on the membrane just before egress, which is achieved by timely discharge of PfPLP1 from merozoites. Furthermore, RBCs treated with rPfPLP1 and rMACPF also show permeabilization as Phalloidin enters and stains rPfPLP1- and rMACPF-treated RBCs. This suggests that PfPLP1 possesses permeabilizing and membranolytic capabilities ( Fig. 6g ). The Ca 2+ dependence of membranolytic activities of rPfPLP1 and rMACPF domain were tested in the presence and absence of EGTA. rPfPLP1 but not rMACPF showed Ca 2+ -dependent membranolytic activity ( Fig. 6c ). In addition to Ca 2+ -dependent membranolytic activity, rPfPLP1 showed Ca 2+ -dependent membrane binding ( Fig. 6h ). The Ca 2+ -dependent membranolytic activity of rPfPLP1 could be due to the presence of β-pleated sheets at its C-terminal domain that is structurally homologous to the C-terminal domain of lymphocyte perforin [52] . Deletion of the C-terminal domain of PfPLP1 did not inhibit its membranolytic activity [51] but abolished its Ca 2+ dependence supporting the fact that the C-terminal region is responsible for conferring its Ca 2+ dependence similar to human perforin [53] . The C-terminal domain of lymphocyte perforin has been shown to be responsible for Ca 2+ -dependent membranolytic activity [39] , [52] . It has previously been shown that lymphocyte perforin forms oligomers upon binding to membrane and migrate at >1,000 kDa in SDS–polyacrylamide gel electrophoresis (SDS–PAGE), indicative of the incorporation of more than 16 monomers into the complexes [29] , [53] . We also investigated the oligomerization of rPfPLP1 under similar conditions. rPfPLP1 formed oligomers upon incubation with human RBCs in the presence of Ca 2+ , suggesting that binding of PfPLP1 monomer to human RBC leads to its oligomerization as reported for human perforin [29] , [53] . Finally, our results support the hypothesis that increase in intracellular Ca 2+ in late schizonts triggers secretion of PfPLP1 from micronemes. After secretion, PfPLP1 binds to the membrane, oligomerizes and permeabilizes the host cell membrane to facilitate egress ( Fig. 7 ). Pore formation by PfPLP1 may directly destabilize membranes leading to egress or act as gateways for additional effector proteins already present in the PV or released during egress. It would be interesting to study the PfPLP1 knockout phenotype but our several attempts to knock-out PfPLP1 remained unsuccessful. The role of PfPLP2 can be also predicted in the egress of merozoites, as it is also expressed in the schizont stage but in our study it is not seen localized either on the RBCM or PVM ( Supplementary Fig. S7 ). However, it does not restrict us from speculating that PfPLP1 and PfPLP2 may have overlapping roles together in egress or a dominant role in the absence of other, which require further detailed study. This work provides mechanistic insights into blood-stage PfPLP1 and its role in permeabilization of host cell during egress of P. falciparum merozoites, thereby opening the door for development of new chemotherapeutic strategies against malaria. This study suggests that Ca 2+ -dependent microneme discharge not only regulates merozoite invasion, as shown previously but is also crucial for merozoite exit. Signalling pathway components that are involved in apical organelle release should therefore serve as attractive drug targets to limit both parasite egress and invasion. In vitro culture of P. falciparum Laboratory strain of P. falciparum , 3D7 was cultured in RPMI 1640 (Invitrogen, USA) supplemented with 27.2 mgl −1 of hypoxanthine (Sigma Aldrich, USA) and 0.5% Albumax I (Invitrogen, USA) using O + RBCs in mixed gas environment (5% O 2 , 5% CO 2 and 90% N 2 ) as described previously [54] and synchronized by sorbitol selection of rings. Live-cell video microscopy during egress To study intracellular Ca 2+ flux, purified P. falciparum schizonts were loaded with Fluo-4AM, placed in coverslip bottom petriplates and observed under a confocal microscope equipped with a temperature-controlled stage (Nikon A1R). DIC and fluorescent images (505–550 bandpass filter) were captured using a × 100, 1.4 numerical aperture lens. 12-bit time-lapse images of egress events were captured. To test host cell membrane permeabilization during egress, purified P. falciparum schizonts were placed in coverslip bottom petriplates along with 100 μM Phalloidin Alexa 594 and observed for rupture of schizonts under confocal microscope. DIC and fluorescent images (590–665 bandpass filter) were captured. Parasite egress and permeabilization assay To assess the effect of Ca 2+ -modulating agents on parasite egress, aliquots of late-stage schizonts (~44–46 h post invasion (hpi)) were diluted to a final haematocrit of 2% and parasitemia of ~10% and treated with 50 μM of BAPTA-AM (Calbiochem, USA), 1 mM EGTA, 10 μM E64 (Sigma, USA) and DMSO in iRPMI in control wells in duplicate. Schizonts were incubated for 4–6 h to allow rupture and stained with either ethidium bromide (10 μg ml −1 ) or with Alexa-Fluor 488 Phalloidin (Invitrogen, USA) at a final concentration of 100 nM and acquired by flow cytometer (FACS Calibur, Becton & Dickinson, USA) using Cell Quest software by scoring 100,000 cells per sample. Samples were analysed using FlowJo software (Tree Star Inc, Ashland) by determining the proportion of FL-2-positive cells representing schizonts. % Egress was calculated as the fraction of schizonts ruptured in treatment and control during the incubation time as compared with the initial number of schizonts at 0 h, using the formula as described below. % Egress was then plotted considering fraction of schizonts ruptured in control as 100% egress. I, initial no. of schizonts; T, no. of schizonts in treatment; C, no. of schizont in DMSO control. For permeabilization assay, the percentage of Phalloidin-positive schizonts were compared in E64- and BAPTA-AM-treated schizonts assuming 100% permeabilization for E64-treated cells. Viability assay To check viability of schizonts under different treatment conditions, schizonts were incubated with DHT (10 μg ml −1 ) for 20 min at 37 °C, washed and analysed by flow cytometry (FACS Calibur, Becton & Dickinson, USA) using Cell Quest software by scoring 100,000 cells per sample. An overlay histogram plot with cell number on y axis and DHT fluorescence (FL-2) on x axis was plotted for treated and untreated parasites along with unstained parasites as control for parasite autofluorescence. Immunoblot analysis of PfPLPs Proteins from cell lysate of P. falciparum blood-stage parasites were separated by SDS–PAGE, transferred to polyvinylidene diflouride membranes and detected by enhanced chemiluminescence kit (Amersham, Piscataway, NJ, USA) following western blot using anti-PfPLP mouse sera at a dilution of 1:200. GST and pre-immune sera were used as negative control. Immunofluorescence assay Methanol-fixed slides of ring, trophozoite and schizont stages of P. falciparum -infected RBC were blocked with 3% BSA in PBS for 2 h at room temperature (RT) and probed with anti-PfPLP1 and anti-PfPLP2 mouse sera diluted 1:100, followed by Alexa-Fluor 488-conjugated goat anti-mouse IgG antibody, diluted 1:200. For co-immunostaining, smears were also probed with anti-EBA-175 (1:50) rabbit sera, anti-CLAG3.1 (1:100) rabbit sera (kindly provided by Dr Osamu Kaneko, Japan) or anti-PfMSP1 19 (1:100) rabbit sera followed by incubation with Alexa-Fluor 488-labelled goat anti-mouse IgG (1:200) and Alexa-Fluor 594 (1:500)-labelled goat anti-rabbit IgG (Molecular Probe, Eugene, OR, USA), for 1 h at RT. The slides were washed and mounted with DAPI antifade mounting media (Molecular Probe, Eugene, OR, USA). For membrane staining of schizonts along with PfPLP1, slides were stained with PKH26 Red Fluorescent Cell Linker Dye (Sigma, USA) for 2 min at RT following PfPLP1 staining and mounted in DAPI antifade mounting media (Molecular Probe, Eugene, OR, USA). For localization of PfPLP1 on the PVM, E64 (10 μM)-treated schizonts were smeared on glass slides and stained for PfPLP1 and band3 (1:50) as described above. The parasites were visualized using Nikon A1R confocal microscope and images were processed by Imaris version 6.4.2 or 7.0.0 (Bitplane Scientific), which provides functionality for the visualization, segmentation and interpretation of 3D microscopy datasets. For clarity of display, deconvolved z stacks were reconstructed in 3D, with interpolation. Immunoelectron microscopy Isolated P. falciparum merozoites were fixed in 2.5% glutaraldehyde (Sigma, USA) for 2 h at 4 °C and washed twice with 0.1 M phosphate buffer (pH 7.2). Merozoites were dehydrated with increasing concentration of electron microscopy-grade ethanol (30, 50, 70, 80, 90 and 100%) and incubated with absolute ethanol and LR White (EMS, USA) in 1:1 ratio for 1 h followed by overnight incubation in LR White at 4 °C. Finally, the sample was embedded in LR White at 55 °C for 24 h and sectioned with a Leica Ultracut UCT cryo-ultramicrotome (Leica Microsystems Inc., Bannockburn, IL). Ultrathin sections were blocked in 2% skimmed milk in double distilled water at RT for 1 h and incubated with anti-PfPLP1 mouse sera in fish gelatin (1:5 dilution) overnight at 4 °C followed by incubation with goat anti-mouse IgG (1:50 dilution in fish gelatin) for 2 h at RT. Stained sections were incubated in saturated solution of uranyl acetate for 3–5 mins at RT and visualized under electron microscope, FEI-Tecnai T12. Secretion assay To analyse the secretion of PfPLP1 from intraerythrocytic merozoites, schizonts (~44–46 hpi) were treated with 1 mM EGTA, 50 μM BAPTA-AM and DMSO control for 4–6 h at 37 °C. PV and RBC fractions of schizonts were collected by 0.05% saponin treatment and probed for the presence of PfPLP1 by western blot analysis using anti-PfPLP1 mouse sera [7] . To analyse secretion of PfPLP1 from free merozoites, merozoites were isolated as described previously [37] and incubated with iRPMI, iRPMI containing 1 mM EGTA, iRPMI containing 50 μM BAPTA-AM and iRPMI containing 4 μM A23187 for 15 min at 37 °C. Following incubation, supernatants were separated by centrifugation and used for detection of PfPLP1 and AMA1 by western blotting using anti-PfPLP1 mouse sera (1:200), anti-AMA1 rabbit sera (1:2,000) or anti-NAPL rabbit sera (1:2,000) followed by horse radish peroxidase (HRP)-conjugated anti-mouse or anti-rabbit IgG goat sera (Sigma, USA). Erythrocyte-binding assay Binding of native PfPLP1 and rPfPLP1 to human RBCs was performed as described previously [55] . Briefly, human RBCs were incubated with collected supernatant of ruptured schizonts or rPfPLP1 for binding at 37 °C for 1 h and layered onto dibutyl pthalate (DBT) and centrifuged. Human RBC-bound proteins were eluted using 1.5 M NaCl and detected by western blotting using anti-PfPLP1 mouse sera. To detect the Ca 2+ -dependent binding of PfPLP1, EBA was performed in the presence and absence of EGTA (1 mM). Expression of recombinant PfPLP1 and lysis assay A codon-optimized synthetic gene encoding full-length PfPLP1 gene (PFD0430c, excluding signal sequence, encoding 26–842 amino acids (aa)) and its MACPF domain (encoding 233–571 aa) were subcloned into mammalian expression vector, pRADU adjacent to the secretory signal sequence. The resultant clones were labelled as PfPLP1-pRADU and MACPF-pRADU. For expression of recombinant protein, rPfPLP1 and rMACPF, mammalian Human Embryonic Kidney 293 cells (HEK-293) cultured in Dulbecco Modified Eagle Medium (DMEM; Invitrogen, USA) with 10% heat-inactivated fetal calf serum in a humidified CO 2 (5%) incubator at 37 °C were transfected with PfPLP1-pRADU and MACPF-pRADU using jetPRIME reagent according to manufacturer’s protocol (Hichem Life Sciences). After 48 h, the supernatant of transfected HEK-293 cells containing secreted protein was harvested and used for purification of rPfPLP1 and rMACPF by Ni-NTA chromatography. The purified rPfPLP1 and rMACPF were analyzed by western blotting and for their functional lytic activities. In the lysis assay, rPfPLP1 and rMACPF were added to 5 × 10 6 human RBCs resuspended in 50 μl of lysis buffer containing 150 mM NaCl, 1 mM CaCl 2 and 20 mM Hepes (pH7.2) and incubated for 30 min at 37 °C. The release of haemoglobin was estimated by measuring absorbance at 405 nm. Cell lysis was expressed as a percentage of maximum haemoglobin release compared with 100% lysis of 5 × 10 6 human RBCs in water. To check the Ca 2+ -dependent lysis of human RBCs, 1 mM EGTA was added to the reaction buffer in place of 2 mM CaCl 2 and lysis assay was performed. Oligomerization of PfPLP1 rPfPLP1 monomer was incubated with human RBCs (5 × 10 6 ) in 50 μl of lysis buffer at 37 °C for 30 min. The HBRCs were immediately chilled on ice, pelleted at 4 °C, resuspended in SDS sample buffer and subjected to step SDS–PAGE with the stack section at 4% (w/v), the top separating section at 6% (w/v) and the bottom separating section at 10% acrylamide, and transferred to nitrocellulose membrane for western blotting with anti-PfPLP1 mouse sera. How to cite this article: Garg, S. et al . Calcium-dependent permeabilization of erythrocytes by a perforin-like protein during egress of malaria parasites. Nat. Commun. 4:1736 doi:10.1038/ncomms2725 (2013).